Loss-of-heterozygosity facilitates passage through Haldane’s sieve forSaccharomyces cerevisiaeundergoing adaptation Haldane's sieve posits that the majority of beneficial mutations that contribute to adaptation should be dominant, as these are the mutations most likely to establish and spread when rare. It has been argued, however, that if the dominance of mutations in their current and previous environments are correlated, Haldane’s sieve could be eliminated. We constructed heterozygous lines of Saccharomyces cerevisiae containing single adaptive mutations obtained during exposure to the fungicide nystatin. Here we show that no clear dominance relationship exists across environments: mutations exhibited a range of dominance levels in a rich medium, yet were exclusively recessive under nystatin stress. Surprisingly, heterozygous replicates exhibited variable-onset rapid growth when exposed to nystatin. Targeted Sanger sequencing demonstrated that loss-of-heterozygosity (LOH) accounted for these growth patterns. Our experiments demonstrate that recessive beneficial mutations can avoid Haldane’s sieve in clonal organisms through rapid LOH and thus contribute to rapid evolutionary adaptation. New mutations theoretically establish in diploid populations with a probability that is proportional to their effect on fitness ( s ) scaled by their dominance coefficient ( h ) [1] . Consequently, more dominant mutations (larger h) are thought to be more likely to contribute to adaptation, a phenomenon known as Haldane's sieve. If adaptation occurs via alleles already present in the population, however, the probability of fixation for newly favourable alleles depends on the dominance of mutations in both their new and previous environments [2] , [3] . In fact, if the dominance of beneficial alleles is perfectly correlated with their dominance in a previous environment (where they were deleterious), then Haldane’s sieve vanishes [2] , [3] . Intuitively, recessive beneficial alleles, while less likely to fix, are more likely to start at higher frequency because their previously deleterious effects were better masked. Whether dominance coefficients are positively correlated in different environments has not, however, been explicitly tested. One study in Arabidopsis thaliana found that for two out of six mutants the dominance class in an unstressful environment (where all homozygous mutations were deleterious) did not correspond with the dominance class identified under herbicide stress (where the mutations were beneficial) [4] . Follow-up work with these two mutants found that the homozygous resistance lines did not decline in frequency across multiple generations in the absence of herbicide [5] , suggesting that they were not actually deleterious and rendering the data more difficult to interpret. Thus, although dominance may well change among environments, further data are required, particularly for newly acquired beneficial mutations that have not had any opportunity for dominance to evolve [6] . A further consideration in the discussion of the fixation of beneficial alleles in asexual diploids is the assumption that rare alleles remain heterozygous. One parental allele may be lost through non-meiotic means due to gene conversion, double or single crossover events during mitosis, nonreciprocal chromosomal events or copy number changes (through local deletion, chromosome loss or global ploidy reduction). The rate of these loss-of-heterozygosity (LOH) events may be high enough to enable asexual diploid populations to adapt at a rate more similar to sexual diploid populations, which are able to bring together beneficial mutations in homozygotes through segregation [7] . LOH has been documented in both long-term in vitro microbial experimental evolution experiments [8] , [9] , [10] , [11] and in clinical fungal strains isolated following antibiotic drug exposure [12] , [13] , [14] . LOH has also been shown to arise during plant breeding [15] and is known to be important in the induction of many cancer types; in particular, individuals carrying non-functional tumour-suppressor alleles in heterozygous form are vulnerable to secondary somatic LOH events that inactivate the wild-type allele [16] , [17] . Despite the importance of dominance and LOH of beneficial mutations to health, adaptation and evolution, we still lack an adequate picture of these phenomena. Here we set out to measure heterozygous fitness in multiple environments for a panel of 20 unique beneficial mutations isolated in Saccharomyces cerevisiae in the presence of the fungicide nystatin [18] . Importantly, as the mutations were acquired in haploids, they represent an unbiased set of mutations with respect to their dominance in diploids. Each line carries a mutation (identified through whole-genome sequencing) in one of four genes that act late in the ergosterol biosynthesis pathway (one mutation each in ERG7 and ERG5 , seven unique mutations in ERG6 and eleven unique mutations in ERG3 ). These mutations confer a large fitness benefit in both haploids [18] and homozygous diploids [19] grown under nystatin stress, and yet bear a fitness cost relative to wild type in YPD (a rich medium composed of yeast extract, peptone and dextrose) [18] . Although the exact ecological history of the strain is unknown, YPD is a commonly used rich medium and we use it to represent a previously experienced and unstressful environment, relative to the novel and stressful environment containing nystatin. Thus, these same mutations can be either beneficial or deleterious, depending on the environment. Through crosses, we generated diploid heterozygous lines, whose fitness was then compared with wild-type and homozygous mutant diploids in both YPD and nystatin. As we know the precise genetic basis of each mutation, we were also able to directly measure the rate of LOH after growth in each environment. We identify no correlation between dominance in the two environments: the mutations exhibit a range of dominance levels in an unstressful medium (standard laboratory YPD, where the mutations are deleterious), yet are exclusively recessive under nystatin stress (where the mutations are beneficial). We do, however, find rampant evidence of LOH when lines are incubated in the presence of nystatin. Thus, while these beneficial mutations in heterozygous form seemingly confer no benefit at the cellular level in nystatin, LOH events were routinely selected and reached high frequency, allowing the populations to exhibit adaptation patterns expected of dominant mutations. Importantly, although dominance in the unstressful, previously experienced environment does not offset dominance in the current nystatin environment, LOH provides a rapid mechanism to enable beneficial mutations that are recessive at the cellular level to reach high frequency, as if they were dominant beneficial mutations at the population level, mitigating the effects of Haldane’s sieve. Dominance is not correlated among environments In an unstressful medium (standard laboratory YPD), we observed a large range of dominance coefficients for growth rate and biomass production measured in a plate reader ( Fig. 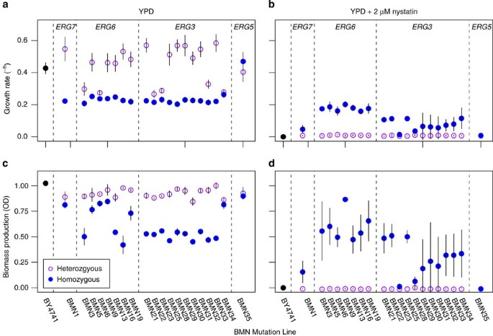Figure 1: Fitness assay of heterozygous and homozygous mutation lines reveals variation in dominance among environments. A comparison among lines for both maximal growth rate (a,b) and biomass production (optical density at 24 h,c,d) indicates that lines with heterozygous mutations (open purple circles) outperform lines with homozygous mutations (closed blue circles) in YPD ((a) growth rate, (c) biomass production) but were not capable of growth in YPD+2 μM nystatin ((b) growth rate, (d) biomass production). Lines on thexaxis are arranged by the gene that carries a mutation; the lines farther to the left carry mutations in genes that are most upstream from the production of ergosterol, the end product of the pathway. When multiple mutations are present within a gene, the lines are arranged from 5′ to 3′ sites within the gene. Error bars reflect the s.e.m.s for each line from experiments conducted on five separate days for YPD and two separate days for nystatin. 1 ; Table 1 ). Owing to variation among replicate experimental days (see Methods) we focus on categorical differences among mutations: recessive if heterozygous fitness was significantly different from the homozygous mutant but not wild type, dominant if heterozygote fitness was significantly different from the wild type but not the homozygote, intermediate if the heterozygote was significantly different and intermediate compared with either and overdominant if the heterozygote grew significantly better than both homozygote and wild type. 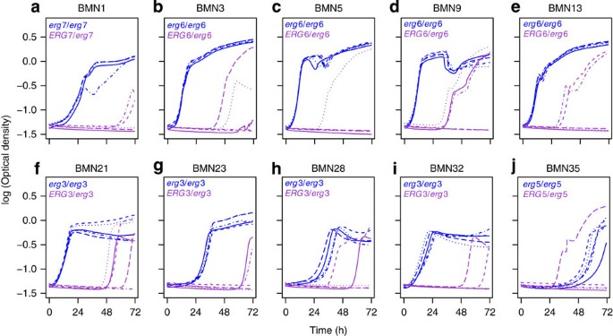Figure 2: Heterozygotes grow stochastically in the presence of nystatin. Homozygous (blue) and heterozygous (purple) mutant diploid lines were grown in YPD+2 μM nystatin. Stochastic growth was observed in all 20 BMN lines (shown here is a representative sample). (a) BMN1, which has a mutation inERG7, (b–e) BMN3, 5, 9 and 13, which contain mutations inERG6, (f–i) BMN21, 23, 28 and 32, which contain mutations inERG3, and (j) BMN35, which has a mutation inERG5. The same initial culture was placed into five replicate wells for each BMN line. Almost half of the fitness assays (45%) indicated that the mutations were recessive in YPD, yet we also identified cases of intermediate fitness (20% of assays, primarily for biomass production), dominance (15% of the assays) and overdominance (7.5% of assays; Table 1 ; 12.5% of assays were inconclusive, full growth rate statistics: Supplementary Table 1 , full biomass production statistics: Supplementary Table 2 ). By contrast, when lines were incubated in YPD+2 μM nystatin or YPD+4 μM nystatin, none of the heterozygous lines exhibited growth within 24 h, by which time the homozygous lines had grown to nearly stationary-phase levels ( Fig. 1 ). Thus, all of the mutations were recessive in nystatin, and there is no correspondence in dominance between the two environments. Figure 1: Fitness assay of heterozygous and homozygous mutation lines reveals variation in dominance among environments. A comparison among lines for both maximal growth rate ( a , b ) and biomass production (optical density at 24 h, c , d ) indicates that lines with heterozygous mutations (open purple circles) outperform lines with homozygous mutations (closed blue circles) in YPD (( a ) growth rate, ( c ) biomass production) but were not capable of growth in YPD+2 μM nystatin (( b ) growth rate, ( d ) biomass production). Lines on the x axis are arranged by the gene that carries a mutation; the lines farther to the left carry mutations in genes that are most upstream from the production of ergosterol, the end product of the pathway. When multiple mutations are present within a gene, the lines are arranged from 5′ to 3′ sites within the gene. Error bars reflect the s.e.m.s for each line from experiments conducted on five separate days for YPD and two separate days for nystatin. Full size image Table 1 Estimated dominance coefficients in YPD for heterozygous lines. Full size table Stochastic growth of BMN lines in the presence of nystatin When we continued growth in the presence of 2 or 4 μM nystatin for longer (up to 72 h), we surprisingly observed stochastic growth of heterozygous replicates ( Fig. 2 ), reminiscent of the growth patterns observed when the haploid ancestor first acquired beneficial mutations [18] . To confirm these results, we tracked growth at 1, 2 and 4 μM nystatin in deep-well boxes, which allowed us to simultaneously assay a much higher number of replicates than in a plate reader. After 72 h of exposure, the majority of heterozygous replicate wells grew to either a similar optical density as homozygous lines or not at all, with the fate varying among replicates within lines ( Fig. 3 ). We subsequently repeated the deep-well experiment ( Supplementary Fig. 1 ) and froze culture from all wells after 36 h (1 μM nystatin) or 80 h (2 and 4 μM nystatin). The proportion of replicates that grew across the two box experiments was significantly influenced by the level of nystatin in the medium as well as the gene bearing the mutation (two way analysis of variance (ANOVA); environment: F 1,112 =54.47, P <0.0001, gene: F 3,112 =4.29, P =0.007, interaction: F 3,112 =2.52, P =0.061). Approximately double the number of replicates grew in lower levels of nystatin (95% of replicates in 1 μM nystatin and 83% of replicates in 2 μM nystatin) compared with the highest level (52% of replicates in 4 μM nystatin). Figure 2: Heterozygotes grow stochastically in the presence of nystatin. Homozygous (blue) and heterozygous (purple) mutant diploid lines were grown in YPD+2 μM nystatin. Stochastic growth was observed in all 20 BMN lines (shown here is a representative sample). ( a ) BMN1, which has a mutation in ERG7 , ( b – e ) BMN3, 5, 9 and 13, which contain mutations in ERG6 , ( f – i ) BMN21, 23, 28 and 32, which contain mutations in ERG3 , and ( j ) BMN35, which has a mutation in ERG5 . The same initial culture was placed into five replicate wells for each BMN line. 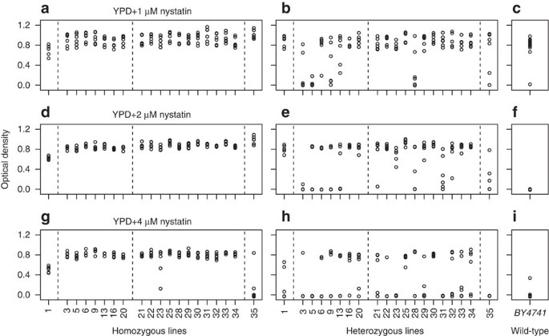Figure 3: Frequency of heterozygous growth in deep-well boxes varies with environment and line. Lines were grown in the presence of (a–c) 1 μM nystatin, (d–f) 2 μM nystatin and (g–i) 4 μM nystatin. Four replicates were measured after 72 h of growth for homozygotes (a,d,g) and heterozygotes (b,e,h) from each line (eight replicates were measured for the wild type (c,f,i)). Compared with the consistent growth of homozygous lines (except BMN23 and BMN35 in 4 μM nystatin, which have the weakest nystatin tolerance), the heterozygous lines typically showed a stochastic pattern with some replicates that grew and some that did not. Full size image Figure 3: Frequency of heterozygous growth in deep-well boxes varies with environment and line. Lines were grown in the presence of ( a – c ) 1 μM nystatin, ( d – f ) 2 μM nystatin and ( g – i ) 4 μM nystatin. Four replicates were measured after 72 h of growth for homozygotes ( a , d , g ) and heterozygotes ( b , e , h ) from each line (eight replicates were measured for the wild type ( c , f , i )). Compared with the consistent growth of homozygous lines (except BMN23 and BMN35 in 4 μM nystatin, which have the weakest nystatin tolerance), the heterozygous lines typically showed a stochastic pattern with some replicates that grew and some that did not. Full size image Rapid LOH in the presence of nystatin We suspected that heritable genetic changes had arisen in the replicates that grew in nystatin. Indeed, when culture from wells that grew were placed back into the stressful medium, growth trajectories were consistent, similar to the homozygous lines ( Supplementary Fig. 2 ). We theorized that LOH at the initial mutation locus could explain the growth observed. We Sanger-sequenced ~1,000 bp around the known mutation in 84 heterozygous replicates, sub-sampled from all lines that showed growth in YPD, YPD+1 μM nystatin, YPD+2 μM and YPD+4 μM nystatin (hereafter referred to as ‘het-grow’ lines, primers listed in Supplementary Table 3 ). 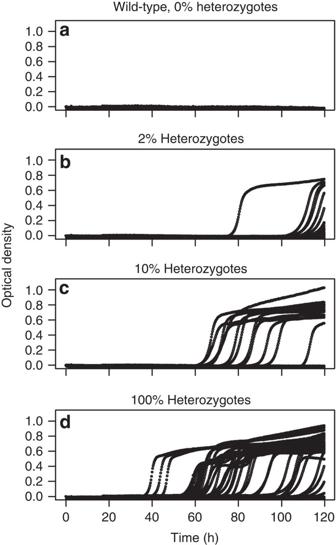Figure 4: Populations containing heterozygotes adapt to nystatin (2 μM) more frequently than those that do not. While none of the populations composed entirely of (a) wild-type cells grew, populations that contain (b) 2, (c) 10 or (d) 100% heterozygotes grow stochastically, indicative of LOH. All 13 het-grow lines isolated after growth in YPD remained heterozygous ( Supplementary Table 4 ). In contrast, in 1 μM nystatin, 25 of 29 het-grow replicates were homozygous for the initial mutation ( Supplementary Table 5 ). The other four lines were all initiated from BMN35 (with a mutation in ERG5 ) and the populations were polymorphic for heterozygous and homozygous mutant diploid individuals, suggesting homozygous diploid mutants were in the process of sweeping through the populations ( Supplementary Fig. 3 ). All het-grow replicates isolated from 2 and 4 μM nystatin lost heterozygosity of the adaptive nystatin mutations ( Supplementary Tables 6 and 7 ). The majority (34/42 lines) became homozygous for the initial ergosterol mutation, although we also found eight replicates that were homozygous wild type at the initial locus ( Supplementary Table 8 ), and yet contained homozygous ergosterol mutations carried by other lines in our screen. These eight cases are consistent with contamination events during the multiple rounds of sampling from the deep-well boxes when isolating the het-grow lines (see Methods) and were not included in the remainder of our analyses. LOH in mixed populations of wild-type and heterozygous cells While LOH may contribute strongly to adaptation of populations initially composed entirely of heterozygous cells (as we have shown), it is more likely that neutral or weakly deleterious heterozygotes generally comprise a minority of a population when it first experiences a novel environment. Exactly what fraction of a population is expected to carry a mutation depends on the nature of selection in the previous environment. Mutation-selection balance predicts that deleterious heterozygotes would be at frequency 2 μ/( h s) for h >0, which is exceedingly small per site (for example, ~6.3 μ for BMN3, based on its growth in YPD) but may become large if many sites can contribute to adaptation. However, many of our mutations were recessive or overdominant in YPD; in both cases the heterozygous frequency should approach one with asexual reproduction. Even in sexual populations, the frequency of deleterious mutations is highly variable. For example, a search for deleterious alleles in the HapMap data set found that almost half were at frequencies >2% while a quarter were at frequencies >50% [20] . We thus repeated our growth rate assays in the plate reader at a number of initial heterozygous frequencies, (0, 2, 10 and 100%) to examine whether LOH events remain prevalent. We found a striking pattern between the appearance of growth and the frequency of heterozygotes in the population ( Fig. 4 ). Although none of the 96 populations with 0% heterozygotes exhibited growth after 120 h in YPD+2 μM nystatin ( Fig. 4a ), when the populations contained 2, 10 or 100% heterozygotes we found that 5, 21 and 60% of wells grew ( Fig. 4b–d ). We thus infer that LOH remains an important source of adaptive genetic change even in populations that initially contain a smaller fraction of heterozygous cells. Figure 4: Populations containing heterozygotes adapt to nystatin (2 μM) more frequently than those that do not. While none of the populations composed entirely of ( a ) wild-type cells grew, populations that contain ( b ) 2, ( c ) 10 or ( d ) 100% heterozygotes grow stochastically, indicative of LOH. Full size image Possible mechanism of LOH LOH can be accomplished by a number of mechanisms, including gene conversion, mitotic recombination and copy number changes. We identified only a single ploidy change through flow cytometry of the 84 het-grow lines: BMN3-188 (a line isolated after growth in 2 μM nystatin) had become haploid. To look for localized copy number changes we whole-genome-resequenced the six lines isolated after growth in YPD+2 μM nystatin that exhibited the lowest G1 mean and conducted genome-wide analyses of the depth of coverage. We saw very few cases of whole-chromosome aneuploidy (none involving the chromosome carrying the relevant ergostergol genes, Supplementary Fig. 4 ) and no cases of partial aneuploidy ( Supplementary Fig. 5 ). We similarly found no evidence for local gene deletion at the level of each ergosterol gene in the sequenced het-grow lines through in silico qPCR (a computational method to count read depth on short representative fragments in the unaligned fastq files, see Methods, Supplementary Fig. 6 ). As our experiments purposefully utilized lines that were generally identical except for the nystatin-adaptive mutations, they did not contain markers that would allow us to quantify crossover events or gene conversion patterns. Approximately half of the lines do, however, carry secondary mutations at some location in the genome ( Supplementary Table 9 , there is no evidence that these mutations contribute to nystatin tolerance [18] ). All secondary mutations remained heterozygous with a single exception. BMN31, with a mutation in ERG3 , carries a secondary mutation in ALT1 located 64 kb distal to ERG3 on chromosome XII; all four resequenced het-grow replicates initiated from BMN31 (two isolated in 1 μM nystatin and two in 4 μM nystatin) were homozygous for the second mutant allele. Altogether, these results are consistent with localized (that is, at most single chromosome) LOH, rather than whole-genome LOH (that is, through ploidy cycles). Interestingly, although mitotic repair of double-stranded breaks by homologous recombination has previously been found to be the most common mechanism enabling LOH in S. cerevisiae [21] , [22] , our results are not consistent with mitotic recombination as the primary mechanism here. The rate of mitotic recombination has been found to increase linearly with distance from the centromere in S. cerevisiae [7] and Candida albicans [11] , yet lines with a mutation in ERG6 , which is only ~15 kb away from its centromere in the reference strain, underwent LOH at a similar rate as lines with a mutation in ERG3 , which is located ~102 kb away from its centromere ( ERG3 is the other gene where we identified multiple mutations and thus is the best comparison). A recent experiment in C. albicans lines found whole-chromosome LOH to be the most frequent mechanism enabling LOH in lines subjected to fluconazole, an antifungal drug similar to nystatin [11] . This mechanism is consistent with the observation that LOH was observed at secondary sites only in BMN31, which carried both ERG3 and ALT1 mutations on the same chromosome. Here we uncovered striking variation in dominance coefficients between two environments: in an unstressful, previously experienced environment (a standard laboratory environment, YPD) where the mutations are deleterious in homozygous diploids, the mutations exhibited a wide range of effects in heterozygous form. In nystatin, the environment in which the mutations were originally acquired, all mutations were recessive, conferring no measurable fitness benefit in the heterozygous state when fitness was assayed over 24 h. This variation in dominance between two environments could be explained in at least two ways. From the perspective of a single pathway, sensitivity to alterations in gene product may depend on the environment, which could affect substrate concentrations and/or enzymatic activity. This reasoning is in line with metabolic theory [23] as well as theories about the interplay between genetic and environmental robustness [24] . Second, changes in dominance across environments might be explained by pleiotropy, if the various pleiotropic effects of a mutation have different impacts on fitness in different environments. With respect to our experiment, heterozygous lines producing moderate levels of ergosterol might be nearly as susceptible to nystatin binding as wild-type cells, explaining the recessivity of resistance, and yet the fitness effects in unstressful medium might depend on the exact nature of the intermediate sterol products and/or the exact level of ergosterol produced and how this affects normal functioning of the cell. Regardless of the explanation, the observation of idiosyncratic dominance relationships across environments makes it clear that a nuanced form of Haldane’s sieve must act upon beneficial mutations. Specifically, Haldane’s sieve should be thought of as acting in two dimensions, depending on the dominance properties in both previous and current environments. Haldane’s sieve will be least effective at eliminating those mutations that were recessive when deleterious and dominant when beneficial; our results suggest that this class of mutations may well exist, as the dominance of mutations in one environment does not necessarily predict its dominance in a second. The variation in dominance among mutations in YPD is intriguing; we found that different mutations in the same gene had different dominance properties—a result that was true for both genes that were the targets of multiple mutations. We also found that the two fitness assays we utilized, growth rate and biomass production (optical density at 24 h) often gave different results. The distribution of dominance coefficients for growth rate was bimodal, with the primary group exhibiting a recessive or overdominant phenotype (that is, heterozygous growth similar to or faster than the wild type), and a second group with a dominant phenotype (similar growth as the homozygous mutant). The variation in dominance for growth rate stems from variation among the heterozygotes, as the homozygous mutants (except the line that carries a mutation in ERG5 ) are very similar. The distribution of dominance coefficients for biomass production was much more uniform. Here the variation for dominance among mutations arose primarily because of differences in biomass production of the homozygous lines. Heterozygous knockout strains for ERG6 , ERG3 and ERG5 have previously been shown to be recessive in YPD in a pooled competition experiment [25] ; thus, we infer that the proteins produced from the mutations that show dominant properties must behave in a manner that is different from the null allele. The dominant mutations do not group together in an identifiable manner—they are neither the same type of change (they include premature stop codons, amino-acid changes, small and large indels [18] ) nor are they clustered within the primary sequence of the genes or within the secondary structure motifs, although the protein structures for these genes have not been resolved. This is the first data set to examine the dominance properties of different beneficial mutations in the same gene; thus, the variation we uncovered is intriguing and may turn out to be a common feature of adaptive mutations. More experimental data on the dominance properties of beneficial mutations are needed to shed light on this phenomenon. Our results demonstrate one mechanism for recessive beneficial alleles to break the constraint imposed by Haldane’s sieve—we uncovered widespread and rapid LOH within 24–72 h in the presence of even low levels of the stressor in which the mutations are beneficial. Thus, although these mutations are recessive at the cellular level (cells that do not undergo LOH are no more tolerant than wild type), LOH enables them to rapidly homozygose and allows adaptation at the population level as if they carried a dominant mutation. Our experiments were all conducted at a very short timescale (72 h) and indicate that LOH can be both rapid and frequent, particularly with large population sizes and strong selection. LOH was not observed after growth in YPD, even in cases where a revertant to wild type would be more fit than the heterozygous mutant line. Although these heterozgyotes grow slower than wild type, in all cases they still reach substantial biomass by 24 h ( Fig. 1 ). Thus, selection for revertant homozygotes produced by LOH would have been much weaker in YPD than it was in nystatin. The rapid appearance and spread of homozygous individuals in heterozygous populations in the presence of nystatin highlights LOH as an important mechanism to enable recessive mutations to establish and spread within clonal populations. Furthermore, these results indicate the potential difficulty in accurately measuring the fitness and dominance of heterozygotes, particularly if researchers do not account for the possibility of LOH. In YPD+2 μM nystatin, for example, multiple lines exhibited full growth by 72 h ( Fig. 3 ; Supplementary Fig. 1 ), and these mutations would typically be labelled as dominant. It was only through sampling multiple replicates at multiple time points (revealing stochastic growth) followed by post-growth sequencing that the truth emerged: these lines were no longer heterozygous. Although few studies have quantified the rate of LOH, the existing data suggest that LOH is more frequent than point mutations [11] , [26] . Indeed, our results indicate that the rate of LOH in 4 μM nystatin is considerably higher than the beneficial mutation rate: the rate of replicate growth in deep-well boxes (a proxy for LOH) was 50% in only 72 h, nearly double the rate of growth observed over 7 days when wild-type haploid lines were exposed to nystatin in an identical experimental setup (where 26.7% of wild-type haploid-inoculated wells grew [18] ). To further investigate the potential for LOH to increase the adaptation rate of a population, we compared growth of diploid wild-type populations, which require de novo mutations to grow in nystatin, to populations that contain either 2 or 10% heterozygotes, where LOH of existing mutations can enable growth. We found that substantially higher proportions of populations were able to adapt within 120 h when initially seeded with heterozygous lines ( Fig. 4 ). Thus, heterozygous beneficial mutations can increase the ability of a population to adapt even when they are initially rare, as the probability of an LOH event is higher than the acquisition of a new (at least partially dominant) beneficial mutation. This effect will be particularly pronounced in environments such as nystatin, where few (if any) dominant beneficial mutations are available, and demonstrates that the effect of Haldane’s sieve (which should eliminate these recessive mutations from the population before they could contribute to adaptation) can be mitigated by LOH. Whether the distribution of dominance coefficients for beneficial mutations in more complex environments is similar to that seen here remains an unresolved question. The rate of LOH was strongly dependent on the environment, with approximately double the number of LOH events at the lower levels of nystatin (1 and 2 μM) compared with the highest level (4 μM). We hypothesize that the lower levels of nystatin permitted greater survival or growth, increasing the chance than an LOH event arose. This explanation is consistent with the lower number of ERG5 replicates that grew compared to other genes (43% of ERG5 replicates compared to 88%, 73% and 81% of ERG7 , ERG6 , and ERG3 replicates, respectively), as the ERG5 mutant line, BMN35, has a much reduced fitness in nystatin relative to other mutations [19] . Surprisingly, poor growth of the heterozygous lines was observed (except in lines that underwent LOH) even in 1 μM nystatin, a level of stressor in which the wild type was generally able to grow ( Fig. 3 ). This underdominance for growth in 1 μM nystatin suggests that heterozygotes may represent the worst case genotype under this condition, bearing the costs of altered membrane sterols without the benefits of resistance. To our knowledge, no other study has systematically characterized the dominance of a large number of newly acquired beneficial mutations across multiple environments. Although the exact distribution of dominance coefficients will depend on the particulars of the environment and the organism, it seems likely that many beneficial mutations will be at least partially recessive, as found for deleterious mutations [27] . If beneficial mutations could not become homozygous in the absence of sex (at least not until secondary mutations occur), the rate of evolution of diploid asexuals would be substantially reduced relative to that of sexual species [28] . Our experiments confirm that LOH provides a mechanism for recessive alleles to break the constraint imposed by Haldane’s sieve, as theoretically predicted [7] . Indeed, LOH should reduce differences in the rate of adaptation between dominant and recessive beneficial mutations, between haploids and diploids, and between sexual and asexual populations, reducing the costs of asexuality [7] . Although the rate of LOH per cell cycle might be low, given the large population sizes of microbes and the strong selection acting, LOH genotypes can reach high frequencies within a very short number of generations. While our work has focused on single-celled yeast, the rapid amplification of cells having undergone LOH provides a useful framework within which to understand similar selection-amplified LOH events in multicellular organisms. In many cancer types such as retinoblastoma, the initial mutation is recessive but rare LOH events become amplified by selection within the individual (‘somatic selection’), through higher rates of proliferation of cancerous cells. In general, LOH allows recessive beneficial mutations to see the light of selection, enabling faster evolution of traits enhancing cellular growth. Mutation acquisition Heterozygous diploids were created from a panel of 20 haploid BMN lines previously described [18] . The mutations were acquired in background BY4741, MATa his3 Δ1 leu2 Δ 0 met15 Δ 0 ura3 Δ 0 , derived from S288c, which is considered to be ‘wild type’ with respect to mutation and recombination rates. To create heterozygous MATa / MATa diploids, we utilized the same method previously described to create MATa / MATa homozygous diploids [19] (heterozygous and homozygous lines were created at the same time). We transformed a single colony from each mutation line with plasmid pB2647 containing LEU2 while an ancestral BY4741colony was transformed with plasmid pB2649 containing URA3 and MAT α (plasmids kindly donated by Dr David Pellman, Harvard Medical School). Single transformed colonies of each line (mutant and wild type) were acquired on −ura/−leu plates, co-inoculated into 200 μl YPD and spotted on YPD plates. We then replica-plated from YPD on −ura, −leu and YPD plates; a single colony that grew only on YPD plates, indicating loss of both plasmids, was selected as the final mutant heterozygous diploid for each line. Each mutant diploid was assayed for ploidy via flow cytometry as a check that the matings were conducted properly, using standard flow cytometry methods [29] . We Sanger-sequenced half the lines to confirm that the expected mutation was heterozygous. Bioscreen experiments We measured fitness by comparing the growth curves of wild type, heterozygous mutants and homozygous mutants in YPD, YPD+2 μM nystatin and YPD+4 μM nystatin using a Bioscreen C Microbiological Workstation (Thermo Labsystems). We chose to use these fitness proxies rather than competitive fitness (for example, through flow cytometry) to enable us to obtain quantitative measures of fitness for the different mutant lines; initial competition assays between wild-type and homozygous mutant lines in nystatin recovered no appreciable wild-type cells, making all the mutant lines appear equivalent. All mutation lines were streaked from culture maintained at −80 °C on a YPD plate and allowed to grow for 72 h. We then picked a single colony and placed it into 10 ml YPD, allowing it to grow overnight. We standardized the optical density of all lines to that of the lowest optical density and innoculated 10 μl of the standardized culture into 1 ml of the environment that was being tested. Diluted culture (150 μl) from each line of interest was then placed into four replicate non-adjacent cells. The Bioscreen automatically measured optical density every 30 min, from which we estimated the maximal growth rate using a spline-fitting procedure described previously [30] . The entire experiment for growth in YPD was replicated on five separate occasions, restreaking from frozen culture each time. Although the growth trajectories were generally very consistent among the multiple wells measured for each line within an experiment, we found considerable variation among the five experiments (as shown by the error bars in Fig. 1 , which reflect the error in trait means among the five experiments). We also ran two bioscreen experiments in both YPD+2 μM nystatin and YPD+4 μM nystatin, again starting from frozen stock. As LOH events were not expected in the first round of experiments, samples from these cultures were not isolated or frozen. All heterozygous wells that showed growth after the second YPD+2 μM bioscreen experiment were streaked to single colony on YPD plates, and we haphazardly froze a single colony from each in 15% glycerol. For all wells that showed growth after the second YPD+4 μM experiment, as soon as the bioscreen run ended we added 150 μl 30% glycerol to all wells that exhibited growth and froze the entire culture. To assess whether heritable genetic changes had arisen in these lines we grew up stock from the frozen cultures in YPD and initiated a bioscreen experiment as before in nystatin medium. Statistical analysis of bioscreen experiments in YPD We found considerably larger variation among results from different experimental days compared with among replicate line measurements within a day. Thus, the entire experiment in YPD was fully replicated on five different days and in all cases statistics were performed on only the mean result observed on each experimental day (thus, we have five data points for each mutation line; averaging across days before calculating the dominance coefficient was performed to reduce the statistical bias that arises when taking ratios of measurements). The fitness of homozygous and heterozgyous diploids was then compared to ascertain the dominance of mutations in YPD (similar calculations were performed for growth in nystatin, below) Owing to the variation among day replicates, however, we caution against over-interpreting our specific estimates of dominance and focus only on results that are repeatable across experimental batches. We statistically compared the maximal growth rate and biomass production (optical density at 24 h) among the three line types (homozygotes, heterozygotes and wild type) using a one-factor ANOVA. Significance ( P <0.05) was determined from a post hoc Tukey test following an ANOVA on the original fitness data from the five replicate experiments (that is, fitness of the heterozygotes was directly compared with the fitness of homozygous mutants and wild types). Deep-well experiments As with the bioscreen experiments, we conducted the deep-well box experiments twice (initiated from independent colonies; experiment 1: Fig. 3 , experiment 2: Supplementary Fig. 1 ), and yet only froze culture from the second experiment. The deep-well experiments were initiated in a similar manner as the bioscreen experiments. In the first experiment, we grew all 20 unique homozygous and heterozygous BMN mutation lines, plus the wild-type (BY4741), while in the second, we grew only the heterozygous BMN lines. In both cases, the culture was streaked from frozen stock on YPD plates and incubated at 30 °C for 72 h. A single colony was then haphazardly chosen and grown overnight in 10 ml YPD. We standardized 200 μl from each line to the lowest optical density and added 400 μl of YPD to this standardized culture to obtain enough stock solution to inoculate all replicate wells. We then added 12 μl of stock solution from each line to 1 ml of medium containing the appropriate stressor in four replicate deep wells. In the first experiment, heterozygous and homozygous replicates were grown in separate boxes to minimize possible contamination; replicates from the same line were never placed beside each other. We used optical density to look for evidence of growth in heterozygous wells. In the first experiment, we assayed culture only at 72 h. In the second, we assayed the optical density of 150 μl well-mixed aliquots from all wells approximately every 24 h on a BioTek microplate reader (BioTek Instruments Inc. Winooski, VT, USA). Culture from boxes containing heterozygous replicates grown in YPD+1 μM nystatin were frozen after 36 h, while boxes containing heterozygotes grown in the presence of YPD+2 μM nystatin and YPD+4 μM nystatin were frozen after 80 h (in each case by adding 100 μl of well-mixed culture from all wells to 100 μl 30% glycerol). Statistics on the rate of growth was determined from the two deep-well experiments (using OD at 72 h from deep-well experiment one, Fig. 3 , and OD at 80 h from deep-well experiment two, Supplementary Fig. 1 ). We calculated the proportion of replicate wells that grew in the two experiments separately, where ‘growth’ is determined by a change in A600 optical density of at least 0.05 from the start of the experiment to the final time point. We used these two numbers for each line to statistically determine the impact of environment and gene on the rate of growth. Sanger sequencing A small amount of freezer stock from 84 heterozygous replicates that had shown growth was inoculated in 20 ml of YPD and was grown overnight for Sanger sequencing. Genomic DNA extractions were performed using standard protocols [31] . We PCR-amplified ~1,000 bp around the mutation locus of interest and purified the PCR product before Sanger sequencing in the forward direction (primer sequences are located in Supplementary Table 3 ). The Ensembl genome browser ( http://www.ensembl.org ) and the Saccharomyces Genome Database ( http://www.yeastgenome.org [32] ) were used to obtain reference genome sequences, and the Clustalw multiple alignment tool from EBI was used for alignment (with default parameters, http://www.ebi.ac.uk/Tools/msa/clustalw2/ ). Sequence Scanner Software (Applied Biosystems) was used to look at the resulting chromatograms. All mutations and sequences were confirmed by alignment and visual inspection of the chromatograms. Contamination of het-grow lines In eight het-grow lines, the original mutation was not found in either heterozygous or homozygous form by Sanger sequencing. We subsequently resequenced these lines for ERG3 and ERG6 , finding that each line was homozygous for another ergosterol mutation previously identified in our experiment ( Supplementary Table 7 ). The potential sources of contamination are different in the bioscreen and deep-well experiments. In the bioscreen experiments (where we found six contaminated lines out of 28 het-grow sequenced lines), heterozygous and homozygous lines were grown beside each other. We thus suspect that a small number of heterozygous wells were contaminated with homozygous culture at the beginning of the experiment. In the deep-well experiments (where we found only two contaminated lines out of 56 sequenced replicate lines), homozygotes and heterozygotes were grown in different boxes, limiting simple contamination (without LOH) as a source of homozygotes. Nevertheless, two cases of homozygosity for the wild-type allele were observed in the YPD+4 μM nystatin deep-well boxes. In each of these cases, there was evidence that a neighbouring well carrying the contaminating ergosterol mutations had undergone LOH and then contaminated the well in question during sampling (boxes were sampled at multiple time points to characterize stochastic growth). This is consistent with the fact that no contamination events were observed in the YPD+1 μM nystatin deep-well boxes, which were only sampled at a single time point. We also considered whether the lines that appeared to be homozygous for their initial ergosterol mutation and that were interpreted as LOH events might represent ‘cryptic’ contamination (that is, contamination from a homozygous diploid that carries the same mutation). Approximately one-third of the het-grow lines carried non-ergosterol heterozygous secondary mutations before our experiments ( Supplementary Table 8 ). Through Sanger sequencing, we found that all lines remained heterozygous for the secondary mutations, arguing against contamination from diploids that were homozygous at the start of the experiment (except for four BMN31 het-grow lines, whose secondary mutations are linked to the initial ergosterol mutation; discussed in the main text). LOH in mixed populations We chose four representative heterozygous mutation lines, one for each unique gene in our panel (BMN1, BMN9, BMN25 and BMN35 with mutations in ERG7 , ERG6 , ERG3 and ERG5 , respectively) to examine in populations composed of both wild-type and heterozygous cultures. Each heterozygous line and the diploid wild-type line were streaked from frozen culture on YPD and were grown at 30 °C for 72 h. A single colony from each heterozygous line and four colonies from the wild-type line were then inoculated into 10 ml YPD and cultured on a rotor at 30 °C for 24 h. Each heterozygous line was then paired with a single wild-type replicate and four populations were created—one composed of 2% heterozygotes and 98% wild-type (by volume), one composed of 10% heterozygotes, and 90% wild-type, one consisting of 100% heterozygous cells and one with 100% wild-type cells. From these 16 master populations, we added 100 μl to 10 ml fresh YPD+2 μM nystatin. One hundred fifty microlitres from each diluted master population were placed into 12 replicate Bioscreen wells and grown on the plate reader by shaking at 30 °C for 120 h (the maximum period of time before medium declines noticeably because of evaporation). The entire experiment was performed twice; as the results from the two experiments are very similar, we have combined them for presentation and analysis. Illumina sequencing het-grow lines To assess the nature of LOH, genomic DNA from six lines that had lost heterozygosity but showed low G1 mean values (measured from flow cytometery) were resequenced in 100-bp paired-end fragments using Illumina’s HighSeq 2000 (BMN3-188, BMN9-12, BMN9-130, BMN13-54, BMN23-144 and BMN28-14). Library preparations followed standard Illumina protocols (2011 Illumina Inc., all rights reserved), with each line uniquely indexed and run together on a lane. The genomic sequence data were processed using Illumina’s CASAVA-1.8.0. The CASAVA program configureBclToFastq.pl was used to convert to fastq and to separate the sequences by index (allowing one mismatched basepair per index). configureAlignment.pl was then used to align each sequence to the yeast reference genome (scergenome.fasta downloaded from the Saccharomyces Genome Database, http://downloads.yeastgenome.org/genomerelease/r64/ ). Finally, configureBuild.pl was used to call single-nucleotide length polymorphisms and indels and to obtain coverage data. Excluding mitochondrial DNA, the average depth of coverage was 60-fold (ranging from 16.5 to 384.8). In silico qPCR To avoid ambiguities because of alignment issues had there been gene loss, we directly counted the number of 100-bp fragments that contained the first or last 18 bp of each ergosterol gene ( ERG7 , ERG6 , ERG3 and ERG5 ) using ‘grep’ to sum counts in the forward and reverse directions and averaging over the total from the beginning and end of the gene in the unaligned fastq files obtained by Illumina sequencing. As this is the bioinformatics equivalent to a qPCR analysis of WGS data, we refer to this technique as in silico qPCR. Accession codes: The sequences of all BMN lines have previously been deposited in the NCBI-SRA database under the accession code PRJNA168423 . How to cite this article: Gerstein, A. C. et al. Loss-of-heterozygosity facilitates passage through Haldane’s sieve for Saccharomyces cerevisiae undergoing adaptation. Nat. Commun. 5:3819 doi: 10.1038/ncomms4819 (2014).